TheCapsasporagenome reveals a complex unicellular prehistory of animals To reconstruct the evolutionary origin of multicellular animals from their unicellular ancestors, the genome sequences of diverse unicellular relatives are essential. However, only the genome of the choanoflagellate Monosiga brevicollis has been reported to date. Here we completely sequence the genome of the filasterean Capsaspora owczarzaki , the closest known unicellular relative of metazoans besides choanoflagellates. Analyses of this genome alter our understanding of the molecular complexity of metazoans’ unicellular ancestors showing that they had a richer repertoire of proteins involved in cell adhesion and transcriptional regulation than previously inferred only with the choanoflagellate genome. Some of these proteins were secondarily lost in choanoflagellates. In contrast, most intercellular signalling systems controlling development evolved later concomitant with the emergence of the first metazoans. We propose that the acquisition of these metazoan-specific developmental systems and the co-option of pre-existing genes drove the evolutionary transition from unicellular protists to metazoans. How multicellular animals (metazoans) evolved from a single-celled ancestor remains a long-standing evolutionary question. To unravel the molecular mechanisms and genetic changes specifically involved in this transition, we need to reconstruct the genomes of both the most recent unicellular ancestor of metazoans and the last common ancestor of multicellular animals. To date, most studies have focused on the latter, obtaining the genome sequences of several early-branching metazoans, which provided significant insights into early animal evolution [1] , [2] , [3] , [4] . However, available genome sequences of close unicellular relatives of metazoans have been insufficient to investigate their unicellular prehistory. Recent phylogenomic analyses have shown that metazoans are closely related to three distinct unicellular lineages, choanoflagellates, filastereans and ichthyosporeans, which together with metazoans form the holozoan clade [5] , [6] , [7] , [8] . Until recently, only the genome of the choanoflagellate Monosiga brevicollis had been sequenced [9] . This genome provided us with the first glimpse into the unicellular prehistory of animals, showing that the unicellular ancestor of Metazoa had a variety of cell adhesion and receptor-type signalling molecules, such as cadherins and protein tyrosine kinases (TKs) [9] , [10] , [11] . However, many transcription factors involved in animal development, as well as some cell adhesion and the majority of intercellular signalling pathways were not found. They were therefore assumed to be both specific to metazoans and largely responsible for development of their complex multicellular body plans [9] , [12] . This view was further reinforced with the recent genome sequence of another choanoflagellate, the colonial Salpingoeca rosetta [13] . However, inferences based on only a few sampled lineages are notoriously problematic, especially in light of the high frequency of gene loss reported in eukaryotic lineages [14] . Clearly, genome sequences from earlier-branching holozoan lineages are needed in order to robustly infer the order and timing of genomic innovations that occurred along the lineage leading to the Metazoa. Here we present the first complete genome sequence of a filasterean, Capsaspora owczarzaki , an endosymbiont amoeba of the pulmonate snail Biomphalaria glabrata [15] and the sister group to metazoans and choanoflagellates [7] , [8] . Recent analyses identified some proteins in Capsaspora crucial to metazoan multicellularity including cell adhesion molecules such as integrins and cadherins, development-related transcription factors, receptor TKs and organ growth control components [16] , [17] , [18] , [19] , [20] , [21] . However, the whole suite of molecules involved in these pathways and other important systems has not to date been systematically analysed. By comparing the Capsaspora genome with those of choanoflagellate and metazoans, we develop a comprehensive picture of the evolutionary path from the ancestral holozoans to the last common ancestor of metazoans. The genome of Capsaspora We sequenced genomic DNA from an axenic culture of Capsaspora owczarzaki ( Fig. 1 ) and assembled the raw reads of approximately 8 × coverage into 84 scaffolds, which span 28 Mb in total. The N50 contig and scaffold sizes are 123 kb and 1.6 Mb, respectively. We predicted 8,657 protein-coding genes, which comprise 58.7% of the genome. Transposable elements make up at least 9.0% of the genome ( Supplementary Figs S1 and S2 , Supplementary Table S1 and Supplementary Note 1 ), a much larger fraction than in M. brevicollis (1%) [22] or the yeast Saccharomyces cerevisiae (3.1%) [23] . 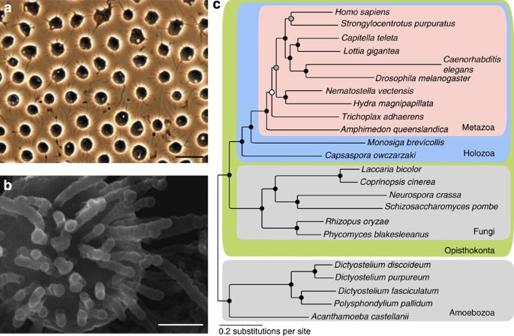Figure 1: The filastereanCapsaspora owczarzaki. (a,b) Differential interference contrast microscopy (a) and scanning electron microscopy (b) images ofC. owczarzaki. Scale bar, 10 μm (a) and 1 μm (b). (c), Phylogenetic position ofC. owczarzaki. Four different analyses on the basis of two independent data sets and two different methods indicate an identical topology, except for the clustering of all non-sponge metazoans (white circle). Details are inSupplementary Note 2. Gray and black circles indicate ≥90% (0.90) and ≥99% (0.99) of bootstrap values and Bayesian posterior probabilities, respectively, for all four analyses. Figure 1: The filasterean Capsaspora owczarzaki. ( a , b ) Differential interference contrast microscopy ( a ) and scanning electron microscopy ( b ) images of C. owczarzaki . Scale bar, 10 μm ( a ) and 1 μm ( b ). ( c ), Phylogenetic position of C. owczarzaki . Four different analyses on the basis of two independent data sets and two different methods indicate an identical topology, except for the clustering of all non-sponge metazoans (white circle). Details are in Supplementary Note 2 . Gray and black circles indicate ≥90% (0.90) and ≥99% (0.99) of bootstrap values and Bayesian posterior probabilities, respectively, for all four analyses. Full size image The Capsaspora genome has a more compact structure than that of M. brevicollis or metazoans, containing 309.5 genes per Mb ( Table 1 ). Genes have an average of 3.8 introns with a mean intron length of 166 bp. The mean distance between protein-coding genes is 724 bp. Interestingly, genes involved in receptor activity, transcriptional regulation and signalling processes have particularly large upstream intergenic regions compared with other genes. ( Supplementary Figs S3–S5 , Supplementary Note 1 ). This pattern is seen across most of the eukaryotic taxa we analysed. In contrast to its compact nuclear genome, Capsaspora has a 196.9 kb mitochondrial genome, which is approximately 12 and 2.6 times larger than the average metazoan mtDNAs (~16 kb) and that of M. brevicollis (76.6 kb), respectively ( Supplementary Fig. S6 , Supplementary Tables S2 and S3 and Supplementary Note 1 ). Our multi-gene phylogenetic analyses with several data sets corroborate that Capsaspora is the sister group to choanoflagellates and metazoans [7] , [8] ( Fig. 1 , Supplementary Figs S7–S10 and Supplementary Note 2 ). Table 1 Genome statistics of Capsaspora owczarzaki and other eukaryotes. Full size table The origins of metazoan protein domains Utilizing all available genome sequences from early-branching metazoans and the two unicellular relatives of the Metazoa ( Capsaspora and M. brevicollis ), we inferred the protein domain evolution along the eukaryotic tree [14] ( Fig. 2 , Supplementary Fig. S11 , Supplementary Tables S4–S7 and Supplementary Note 3 ). We observed a continuous emergence of new protein domains (domains without statistically significant homologies to any proteomes in the outgroup taxa) in the lineage leading to the Metazoa, but also substantial domain loss in fungi, Capsaspora and M. brevicollis . Protein domains acquired by the last common ancestor of filastereans, choanoflagellates and metazoans were enriched in ontology terms associated with signal transduction and transcriptional regulation ( Fig. 2b , Supplementary Table S5 ). Interestingly, such domains include those composing proteins that are involved in metazoan multicellularity and development; for example the cell adhesion molecule integrin-β, and the transcription factors p53 and RUNX ( Fig. 2b , Supplementary Table S4 ). Several domains involved in transcriptional regulation were secondarily lost in M. brevicollis ( Fig. 2c , Supplementary Table S6 ) [17] . Domains involved in extracellular functions have been frequently lost in both Capsaspora and M. brevicollis . Our data indicate that 235 new domains emerged after the divergence of filastereans and choanoflagellates from the lineage leading to the Metazoa. These ‘metazoan-specific innovations’, narrowed down from 299 to 235 by the use of Capsaspora genome, include those that are part of extracellular ligands and their associated components and are involved in metazoan development, such as Noggin, Wnt and transforming growth factor β ( Supplementary Table S4 ). At the root of the Metazoa, we observed significant gains in ontology terms associated with transcriptional regulation and extracellular domains. This ‘metazoan-origin’ domain set, which is much better delineated through comparative analysis using both the Capsaspora and M. brevicollis genomes, likely comprises the key innovations relevant to the evolution of complex multicellular development. 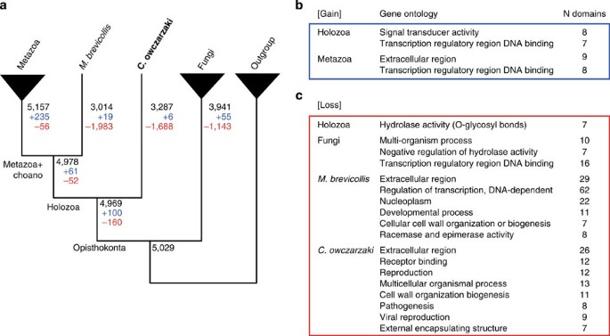Figure 2: Gain and loss of protein domains within the Opisthokonta. (a) The number of Pfam protein domains that were gained or lost at each evolutionary period was inferred by Dollo parsimony, which does not consider multiple independent evolution of a domain. Total number of protein domains, and the inferred numbers of domain gain (+) and loss (−) events are depicted at the tree edges. The full list of domains is inSupplementary Table S4. (b,c) GO terms that were enriched by the evolution of protein domains (b) or depleted by the loss of protein domains (c) were sought via the topology-weighted algorithm. The significant GO terms (P<1.0e−3) are shown at the tree edges together with the number of included Pfam domains. Terms including fewer than seven gained or lost domains are not shown. The list of domains included in each GO is inSupplementary Tables S5 and S6. Figure 2: Gain and loss of protein domains within the Opisthokonta. ( a ) The number of Pfam protein domains that were gained or lost at each evolutionary period was inferred by Dollo parsimony, which does not consider multiple independent evolution of a domain. Total number of protein domains, and the inferred numbers of domain gain (+) and loss (−) events are depicted at the tree edges. The full list of domains is in Supplementary Table S4 . ( b , c ) GO terms that were enriched by the evolution of protein domains ( b ) or depleted by the loss of protein domains ( c ) were sought via the topology-weighted algorithm. The significant GO terms ( P <1.0e−3) are shown at the tree edges together with the number of included Pfam domains. Terms including fewer than seven gained or lost domains are not shown. The list of domains included in each GO is in Supplementary Tables S5 and S6 . Full size image Enrichment of domains in Holozoa Gene duplication is an important evolutionary driving force that increases the functional capacity of proteomes [24] . We thus examined not only the origin of domains involved in metazoan multicellularity but also the abundance of these domains in the genomes of different eukaryotic lineages. We chose 106 InterPro [25] protein domains that are most significantly overrepresented in metazoan genomes compared with the non-holozoan genomes, and counted the number of genes encoding these domains ( Fig. 3 , Supplementary Figs S12 and S13 and Supplementary Note 4 ). Our data show that these domains are, in metazoans, mainly involved in cell adhesion, intercellular communication, signalling, transcriptional regulation and apoptosis, which are relevant to multicellularity and development of metazoans. Most of these domains show clear enrichment exclusively in metazoans. However, the abundance of some of these domains is also increased in the genome of Capsaspora . Those that are particularly enriched include the laminin-type epidermal growth factor-like, Integrin-β4, Sushi, protein tyrosine kinase, Pleckstrin homology, Src homology 3, p53-like transcription factor DNA binding and Band4.1 domain and leucine-rich repeat. These domains are not always similarly enriched in the M. brevicollis genome, as seen, for example, in the Integrin-β4 domain and LRR. Overall, our analyses show that protein domains involved in cellular signal transduction and, to a certain extent, cell adhesion and extracellular regions were already abundant in the common ancestor of the Holozoa, whereas those in other categories such as channels and transporters expanded much later, during metazoan evolution. 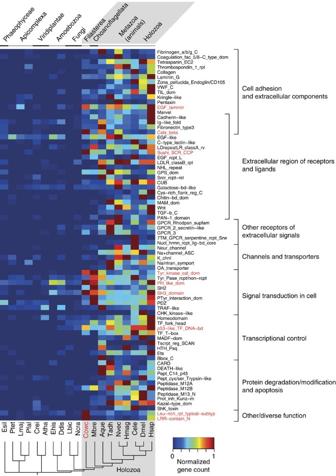Figure 3:Capsaspora owczarzakienrichment of metazoan-biased protein domains. The number of genes encoding proteins that contain each of the selected InterPro domains were analysed (the InterPro short names are shown on the right) for 19 eukaryote genomes. We chose 106 domains that are significantly (Fisher’s exact test;P<1.0e−20) enriched in the metazoan genomes compared with the genomes of non-holozoan lineages. Redundant domains are not exhaustively shown. Domains present only in a single taxon are not shown (available inSupplementary Fig. S12). Values were normalized by the number of all protein-coding genes in the genomes, and relative values to the maximum were calculated. Numbers were manually entered for the protein tyrosine kinase catalytic domain (Tyr_kinase_cat_dom) to exclude mispredicted serine/threonine kinase domains (seeSupplementary Note 5). Protein domains were manually classified into 12 functional categories, shown on the right. In this figure, the categories ‘Zinc-fingers’, ‘cytoskeleton and its control’, ‘Functions on DNA or RNA molecules’, ‘Virus and transposons’ and ‘Other/diverse functions’ are collapsed (only leucine-rich repeats are shown; full figure available in theSupplementary Fig. S13). Domains with high relative gene counts (>0.65) inCapsasporaare depicted in red. Hsap,H. sapiens; Dmel,D. melanogaster; Cele,C. elegans; Hmag,H. magnipapillata; Nvec,N. vectensis; Tadh,T. adhaerens; Aque,A. queenslandica; Mbre,M. brevicollis; Cowc,C. owczarzaki; Ncra,N. crassa; Lbic,L. bicolor; Ddis,D. discoideum; Ehis,E. histolytica; Atha,A. thaliana; Crei,C. reinhardtii; Pfal,P. falciparum; Lmaj,L. major; Ptet,P. tetraurelia; Esil,E. siliculosus. A widely-accepted phylogeny among species is depicted on the bottom. Figure 3: Capsaspora owczarzaki enrichment of metazoan-biased protein domains. The number of genes encoding proteins that contain each of the selected InterPro domains were analysed (the InterPro short names are shown on the right) for 19 eukaryote genomes. We chose 106 domains that are significantly (Fisher’s exact test; P <1.0e−20) enriched in the metazoan genomes compared with the genomes of non-holozoan lineages. Redundant domains are not exhaustively shown. Domains present only in a single taxon are not shown (available in Supplementary Fig. S12 ). Values were normalized by the number of all protein-coding genes in the genomes, and relative values to the maximum were calculated. Numbers were manually entered for the protein tyrosine kinase catalytic domain (Tyr_kinase_cat_dom) to exclude mispredicted serine/threonine kinase domains (see Supplementary Note 5 ). Protein domains were manually classified into 12 functional categories, shown on the right. In this figure, the categories ‘Zinc-fingers’, ‘cytoskeleton and its control’, ‘Functions on DNA or RNA molecules’, ‘Virus and transposons’ and ‘Other/diverse functions’ are collapsed (only leucine-rich repeats are shown; full figure available in the Supplementary Fig. S13 ). Domains with high relative gene counts (>0.65) in Capsaspora are depicted in red. Hsap, H. sapiens ; Dmel, D. melanogaster ; Cele, C. elegans ; Hmag, H. magnipapillata ; Nvec, N. vectensis ; Tadh, T. adhaerens ; Aque, A. queenslandica ; Mbre, M. brevicollis ; Cowc, C. owczarzaki ; Ncra, N. crassa ; Lbic, L. bicolor ; Ddis, D. discoideum ; Ehis, E. histolytica ; Atha, A. thaliana ; Crei, C. reinhardtii ; Pfal, P. falciparum ; Lmaj, L. major ; Ptet, P. tetraurelia ; Esil, E. siliculosus . A widely-accepted phylogeny among species is depicted on the bottom. Full size image Gene repertoire of Capsaspora To further investigate the evolutionary origin of the molecular components required for multicellularity, we performed homology searches and, in most cases, phylogenetic analyses of genes involved in cell adhesion, transcriptional regulation, cell signalling, and nervous system function ( Supplementary Note 5 ). Additionally, to better understand the basic biology of Capsaspora , we analysed gene families proteins involved in meiosis, cell cycle regulation, flagellum formation, post-transcriptional regulation and small RNA synthesis and functioning. 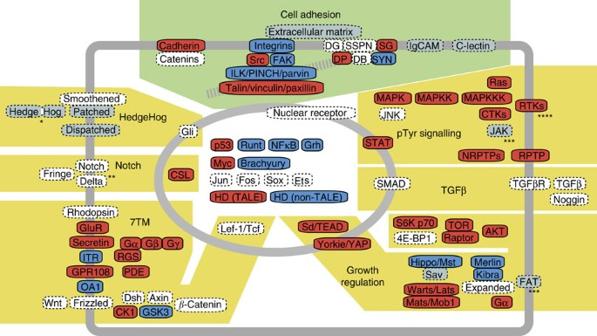Figure 4: Schematic representation of the putativeCapsaspora owczarzakicell. Protein components of major metazoan cell adhesion complexes (green background) and various signalling pathways including receptors (yellow background) are depicted. Components with red and blue backgrounds indicate those found both inC. owczarzakiandM. brevicollisand those found inC. owczarzakibut not inM. brevicollis, respectively. Dotted components are absent in theC. owczarzakigenome; greyed whenM. brevicollishas them. A grey striped line represents an actin filament, to which the cell–ECM–adhesion complexes bind. SeeSupplementary Note 5for details. *, two domains hedge and hog are found in different proteins inM. brevicollis. **, receptor-type proteins with domain architectures similar to Notch and Delta proteins are present inC. owczarzaki. ***, proteins with similar domain architectures are present inM. brevicollis, but not confidently mapped to those metazoan families by phylogenetic analyses. ****, the repertoires of RTKs are totally different betweenC. owczarzaki,M. brevicollisand metazoans, and thus likely to have diversified independently in each lineage. 4E-BP1, eukaryotic initiation factor 4E-binding protein 1; CK1, Casein kinase 1; C-Lectin, C-type lectin; CSL, CBF1/RBP-Jκ/suppressor of hairless/LAG-1; CTKs, cytoplasmic tyrosine kinases; DB, Dystrobrevin; DG, Dystroglycan; DP, Dystrophin; Dsh, Dishevelled; Ets, E-twenty six; FOX, Forkhead box; Gα, G-protein-α subunit; GluR, glutamate receptor; GPR108, G-protein-coupled receptor 108; GSK3, glycogen synthetase kinase 3; Grh, Grainy head; HD, homeodomain; IgCAM, Immunoglobulin-like cell adhesion molecule; ILK, Integrin-linked kinase; ITR, intimal thickness-related receptor; JNK, c-Jun N-terminal kinase; NRPTPs, non-receptor protein tyrosine phosphatases; OA1, Ocular albinism 1-like; PDE, phosphodiesterase; RGS, regulator of G-protein signalling; RTKs, receptor tyrosine kinases; RPTP, receptor protein tyrosine phosphatase; S6K p70; 70kDa ribosomal protein S6 kinase; SAV, Salvador; Sd, Scalloped; SG, Sarcoglycan; SSPN, Sarcospan; SYN, Syntrophin; TALE, three amino-acid loop extension-class homeodomain; TGFβ, Transforming growth factor β; TOR, Target of rapamycin; YAP, Yes-associated protein. Figure 4 schematically summarizes our main findings, depicting the cellular structures and pathways present in Capsaspora and metazoans. We note that none of the analyses provided any evidence of lateral gene transfer events from metazoans to Capsaspora. Figure 4: Schematic representation of the putative Capsaspora owczarzaki cell. Protein components of major metazoan cell adhesion complexes (green background) and various signalling pathways including receptors (yellow background) are depicted. Components with red and blue backgrounds indicate those found both in C. owczarzaki and M. brevicollis and those found in C. owczarzaki but not in M. brevicollis , respectively. Dotted components are absent in the C. owczarzaki genome; greyed when M. brevicollis has them. A grey striped line represents an actin filament, to which the cell–ECM–adhesion complexes bind. See Supplementary Note 5 for details. *, two domains hedge and hog are found in different proteins in M. brevicollis . **, receptor-type proteins with domain architectures similar to Notch and Delta proteins are present in C. owczarzaki . ***, proteins with similar domain architectures are present in M. brevicollis , but not confidently mapped to those metazoan families by phylogenetic analyses. ****, the repertoires of RTKs are totally different between C. owczarzaki , M. brevicollis and metazoans, and thus likely to have diversified independently in each lineage. 4E-BP1, eukaryotic initiation factor 4E-binding protein 1; CK1, Casein kinase 1; C-Lectin, C-type lectin; CSL, CBF1/RBP-Jκ/suppressor of hairless/LAG-1; CTKs, cytoplasmic tyrosine kinases; DB, Dystrobrevin; DG, Dystroglycan; DP, Dystrophin; Dsh, Dishevelled; Ets, E-twenty six; FOX, Forkhead box; Gα, G-protein-α subunit; GluR, glutamate receptor; GPR108, G-protein-coupled receptor 108; GSK3, glycogen synthetase kinase 3; Grh, Grainy head; HD, homeodomain; IgCAM, Immunoglobulin-like cell adhesion molecule; ILK, Integrin-linked kinase; ITR, intimal thickness-related receptor; JNK, c-Jun N-terminal kinase; NRPTPs, non-receptor protein tyrosine phosphatases; OA1, Ocular albinism 1-like; PDE, phosphodiesterase; RGS, regulator of G-protein signalling; RTKs, receptor tyrosine kinases; RPTP, receptor protein tyrosine phosphatase; S6K p70; 70kDa ribosomal protein S6 kinase; SAV, Salvador; Sd, Scalloped; SG, Sarcoglycan; SSPN, Sarcospan; SYN, Syntrophin; TALE, three amino-acid loop extension-class homeodomain; TGFβ, Transforming growth factor β; TOR, Target of rapamycin; YAP, Yes-associated protein. Full size image The unicellular common ancestor of metazoans and Capsaspora appears to have been well equipped with some type of cell adhesion mechanism ( Fig. 4 , Supplementary Fig. S14 , Supplementary Note 5 ). For example, the main components of the integrin adhesion machinery, which in metazoans is used for the attachment of cells to the extracellular matrix (ECM), are present in Capsaspora [16] . However, M. brevicollis lacks integrins and thus choanoflagellates may have secondarily lost them. Even though Capsaspora has integrins, it lacks homologues of metazoan ECM proteins such as fibronectins and laminins. Nevertheless, several protein domains found in these ECM proteins are present as components of other proteins, raising the possibility of unknown ECM molecules secreted by Capsaspora that could interact with its integrin machinery. In contrast to Capsaspora , M. brevicollis , which lacks integrins, has some ECM proteins ( Supplementary Fig. S14 , Supplementary Note 5 ). Capsaspora also has several components of the dystrophin-associated glycoprotein complex, another cell–ECM adhesion system. Both Capsaspora and choanoflagellates have cadherin domain-containing proteins, but M. brevicollis has a much larger repertoire (23 proteins) [9] than Capsaspora , which has only one [21] ( Supplementary Fig. S15 ). Both immunoglobulin-like cell adhesion molecules and C-type lectins, which are lacking in Capsaspora , were present in the unicellular common ancestor of metazoans and choanoflagellates, as they are encoded by the M. brevicollis genome. Several transcription factors arose and diversified in metazoans (for example, those involved primarily in developmental patterning and cell differentiation such as group A basic helix–loop–helix, ANTP-class homeodomains, POU-class homeodomains, Six, LIM, Pax and group I Fox). However, many other transcription factors, including some previously thought to be metazoan-specific, for example, NFκ, RUNX and Brachyury, were already present in the ancestral unicellular holozoans [17] ( Supplementary Figs S16–S18 , Supplementary Table S8 , Supplementary Note 5 ). Interestingly, some transcription factors that act downstream of some signalling pathways in metazoans, such as CSL (Notch–Delta pathway) and STAT (Jak–STAT pathway), are present in Capsaspora , whereas their upstream proteins are missing. Our data reveal the contrasting evolutionary histories of extracellular (or membrane-bound) components versus cytoplasmic components of signalling pathways involved in metazoan multicellularity and development. Most metazoan receptors and diffusible ligands are either ancestral metazoan innovations or have independently diversified in metazoans, whereas the majority of their intracellular components were already present in the unicellular ancestors of metazoans ( Fig. 4 ). Both Capsaspora and M. brevicollis lack receptors and ligands in several systems involved in cell communication and development in metazoans, for example, those in the Hedgehog, Rhodopsin family G-protein-coupled receptors, Wnt, transforming growth factor-β and nuclear receptor signalling pathways ( Fig. 4 ). Notch signalling also seems to be a metazoan innovation, although Capsaspora has several receptor proteins that resemble the metazoan Notch and Delta proteins in their domain architecture, which may represent the ancestral components of this system ( Supplementary Figs S19–S21 , Supplementary Note 5 ). Both Capsaspora and M. brevicollis have large numbers of TKs (92 and 128, respectively) [20] ( Supplementary Figs S22 and S23 , Supplementary Table S9 ). Again, the receptor-type TKs independently diversified in Capsaspora , M. brevicollis and metazoans, whereas the cytoplasmic TKs are mostly homologous among these three lineages, highlighting the animal-specific adaptation of the receptor-ligand system in the Metazoa [20] . The mitogen-activated protein kinase pathway, a downstream cytoplasmic signalling system of the TK pathway, is also present in Capsaspora in the diversified form that we see now in metazoans ( Supplementary Figs S24 and S25 , Supplementary Note 5 ). The diverse members of the G-protein α-subunit family and the regulator of G-protein-signalling family, which together coordinate signal transduction from the 7TM receptors to their specific effectors, are also present in the Capsaspora genome, indicating that the diversity of these components has been secondarily lost, to some extent, in the lineage leading to M. brevicollis ( Supplementary Figs S26 and S27 , Supplementary Note 5 ). Neither sexual reproduction nor meiosis has been reported in Capsaspora . Nonetheless, we identified in its genome a rich repertoire of proteins known to be involved in sex and meiosis in metazoans ( Supplementary Fig. S28 , Supplementary Note 5 ), suggesting the presence of a full sexual reproductive cycle in this organism. Capsaspora also has a rich repertoire of genes involved in cell cycle regulation ( Supplementary Fig. S29 ), including some genes not present in M. brevicollis , such as cyclin E. We also found, as expected, that Capsaspora , which lacks flagellum or cilia, retains only a minor fraction (29 out of 117 genes) of the gene set encoding flagellar components ( Supplementary Fig. 30 , Supplementary Note 5 ). Moreover, all motor protein kinesins, which are involved in various basic cellular functions such as mitosis and transport in many cellular structures, are conserved between Capsaspora and H. sapiens , except for a few families including kinesins 2, 9, 13 and 17, which are thought to be flagellum components [26] . We also identified several RNA-binding proteins ( Supplementary Figs S31 and S32 , Supplementary Note 5 ), some of which are homologous to those involved in stem cell or germ-line cell development, such as bruno, daz, pl10 and pumilio. Although we identified putative homologues of some RNA-binding proteins involved in synthesis and functioning of the non-coding RNA in metazoans (for example, armitage, exportin-5 and Tudor-SN), many other key players (piwi, argonaute, dicer, drosha and pasha) are absent, suggesting either that the non-coding RNA system is non-functional in Capsaspora , or that the silencing mechanism of this filasterean is highly divergent. The Capsaspora genome also possesses, similar to the M. brevicollis genome, a large number of proteins homologous to those involved in neurosecretion and pre- and post- synapse formation and function ( Supplementary Figs S33–S36 , Supplementary Note 5 ). We have reported the first whole genome sequence of a filasterean, a close relative of metazoans. We show that the genome of Capsaspora encodes many proteins that are involved in cell adhesion, signalling and development in metazoans. Previously, the absence of a number of these proteins in the choanoflagellate M. brevicollis and in any sequenced fungi had misled inferences that they were metazoan-specific [12] , [27] , [28] , underscoring the importance of taxonomic sampling in comparative genomics. By adding the whole genome information of the filasterean Capsaspora , the sister group of choanoflagellates and metazoans, we have reconstructed a more robust picture of the unicellular ancestry of metazoans. This evolutionary scenario will be increasingly clarified as genome data from additional holozoan taxa (for example, ichthyosporeans) become available. Our data show that the unicellular common ancestor of metazoans, choanoflagellates and filastereans already possessed a wide variety of gene families that, in metazoans, are involved in multicellularity and development. This early genetic complexity raises at least two possibilities with regard to the ancestral roles of the encoded proteins. First, these proteins may have been already fulfilling functions similar to their roles in extant multicellular animals, such as communication between individual cells and cell-type differentiation. Alternatively, these proteins had different functions such as environmental sensing and later were co-opted for different functions in the multicellular context during metazoan evolution. As cell-cell communication and clear spatial differentiation have not been reported in Capsaspora , the latter possibility seems more plausible. Our analyses of the Capsaspora genome have also more precisely defined the set of proteins and domains that evolved immediately after the divergence of metazoan lineages from filastereans and choanoflagellates. Among those, the evolution of protein components that are involved in intercellular communication represents an especially important step for the innovation of multicellularity. We propose that the acquisition of these new ‘metazoan-specific’ genes with novel functions and the co-option of pre-existing genes that evolved earlier in the unicellular holozoan lineage together represent key innovations that led to the emergence of metazoans. The genome of Capsaspora also opens the door to new research avenues, namely the analysis of the ancestral functions of these genes, which will provide further insights into the molecular mechanisms that allowed unicellular protists to evolve into multicellular animals. Cell culture and nucleic acid extraction and sequencing Live cultures of Capsaspora owczarzaki (ATCC30864) and Ministeria vibrans (ATCC5019; used only for mtDNA sequencing) were maintained at 23 °C in the ATCC 803 M7 medium, and 17 °C in the ATCC 1525 medium, respectively. Genomic DNA and total RNA were extracted using standard methods. Mitochondrial genome MtDNA was sequenced from a random clone library [29] and gaps were filled by sequencing of respective PCR-amplified regions. Gene annotation of the mitochondrial genome was performed with MFannot ( http://megasun.bch.umontreal.ca/cgi-bin/mfannot/mfannotInterface.pl ), followed by manual inspection and addition of missing gene features. Genome sequencing and assembly Genomic DNA was sheared and cloned into plasmid (4 kb pOT and 10 kb pJAN) and fosmid (40 kb EpiFOS) vectors by standard methods. Resulting whole genome shotgun libraries were sequenced by Sanger chemistry, generating approximately eightfold paired-end raw reads: sixfold from the 4 kb library, 1.6-fold from the 10 kb library and 0.8-fold form the 40 kb library. Raw read sequences were submitted to NCBI’s Trace Archive and can be retrieved with the search parameters CENTER_NAME=‘BI’ and CENTER_PROJECT=‘G941’. Sequencing reads were assembled by the Arachne assembler [30] using the default parameters. After assembly, the AAImprover module (part of the Arachne assembler package) was run to improve assembly accuracy and contiguity. Finally, portions of the genome, which appeared to be misassembled, were manually broken to create the final assembly. The assembly was submitted to NCBI with accession number ACFS01000000, BioProject ID PRJNA20341. RNA sequencing Total RNA was isolated from two differently-staged C. owczarzaki cultures with Trizol (Life Technologies). Libraries were sequenced using GAII and HiSeq 2000 instruments (Illumina), which generated 76 base paired-end reads. The RNA-seq data were used for the protein prediction. Gene prediction An initial protein-coding gene set was called with EvidenceModeler [31] by the combination with three ab initio predictions by GeneMark.hmm-ES [32] , Augustus [33] , GlimmerHMM [34] , two sequence-homology-based predictions by Blast and GeneWise [35] and transcript structures built from ESTs by PASA package [36] . The initial gene set was further improved by an incorporation of RNA-seq data using PASA [36] and Inchworm [37] pipelines to obtain a final gene set. Synteny We performed a synteny conservation analysis between C. owczarzaki and M. brevicollis , A. queenslandica and N. vectensis using DAGchainer [38] with default parameters. Phylogenetic analysis We analysed two independent data sets based on whole genome sequences: the mutual best hit (fMBH) data set used for assessing the phylogenetic position of the sponge A. queenslandica [3] and the data set containing 145 putatively orthologous proteins (145POP data set), which were chosen by OrthoMCL2 software [39] . The collected protein sequences were aligned using the MAFFT program [40] , manually inspected and trimmed by the use of Gblocks program [41] with the default parameters. We inferred the maximum likelihood trees by using RAxML 7.2.8 (ref. 42 ) with the LG+Г model. A nonparametric bootstrap test with 100 replicates for each topology was performed. We further tested topologies by the Bayesian inference using PhyloBayes 3.2 (ref. 43 ) with the CAT+Г evolutionary model [44] . The Monte Carlo Markov Chain sampler was run for 10,000 generations, and then burned-in the last 8,000 saving every 10 generations. Protein domain gain and loss analysis We ran the Hmmscan program from HMMER 3.0 package [45] against the Pfam-A version 25 database using protein sets from 35 species: Amphimedon queenslandica, Arabidopsis thaliana, Aspergillus oryzae, Branchiostoma floridae, Brugia malayi, Caenorhabditis elegans, Capitella teleta, Capsaspora owczarzaki, Chlamydomonas reinhardtii, Coprinopsis cinerea, Cryptococcus neoformans, Daphnia pulex, Dictyostelium discoideum, Drosophila melanogaster, Homo sapiens, Hydra magnipapillata, Laccaria bicolor, Lottia gigantea, Monosiga brevicollis, Naegleria gruberi, Nematostella vectensis, Neurospora crassa, Physcomitrella patens, Phytophthora sojae, Rhizopus oryzae, Schizosaccharomyces pombe, Strongylocentrotus purpuratus, Tetrahymena thermophila, Thalassiosira pseudonana, Tribolium castaneum, Trichoplax adhaerens, Trypanosoma brucei, Tuber melanosporum, Ustilago maydis and Volvox carteri. Hits with the scores above the gathering threshold values were considered significant. Dollo parsimony criterion was used to infer the Pfam domains gained and lost along the branches of the phylogenetic tree. The Pfam domains were mapped to GO terms by the use of the Pfam2GO mapping (July 2011). The Ontologizer 2.0 program [46] was used for the GO term enrichment analysis. We evaluated whether a GO functional category evolved in a certain evolutionary position using a P -value calculated by the topology-weighted algorithm [47] . Domain enrichment analysis Protein sets for 12 genomes ( H. sapiens, D. melanogaster, C. elegans, H. magnipapillata, N. vectensis, T. adhaerens, A. queenslandica, M. brevicollis, C. owczarzaki, N. crassa, L. bicolor and D. discoideum ) were first filtered by removing short proteins less than 30 amino acids. For genes that have multiple alternatively spliced isoforms, only the longest protein product was retained for each gene. Protein domain search was performed by the use of InterProScan [48] against InterPro database [25] . The InterProScan results on the complete proteomes of other eukaryotes ( E. histolytica, A. thaliana, C. reinhardtii, P. falciparum, L. major, P. tetraurelia, and E. siliculosus ) were retrieved from the Uniprot ( http://www.uniprot.org/ ) database. Protein domains that are enriched in metazoans compared with all the other non-metazoans except C. owczarzaki and M. brevicollis were selected by the use of Fisher’s exact test ( P <1.0e−20). The number of genes containing such domains, but not the number of domains themselves, was considered. Values were normalized by the numbers of the protein-coding genes in the whole genome. The results were depicted in a heatmap by the R and its Bioconductor package [49] . Intergenic distance analysis We approximated the intergenic distance by calculating the distance between two protein-coding sequences. We then ran two sided t -tests on these distances at upstream (or downstream) regions of genes in each functional category against all other genes in the same genome. Genes were classified by Gene Ontology (GO) [50] annotations, which were generated by the use of Blast2GO [51] and InterPro2GO [52] pipelines. Gene family analysis We chose several gene families that are particularly interesting in the context of the evolution of multicellularity. For each gene family, we inferred the presence and absence of the gene or protein domains in chosen taxa using the HMMER [45] package, mutual Blast and phylogenetic analyses based on maximum likelihood trees inferred by RAxML [42] . Analysed taxa include three bilaterians ( Homo sapiens, Strongylocentrotus purpuratus and Drosophila melanogaster ), three non-bilaterian metazoans ( Nematostella vectensis, Trichoplax adhaerens and Amphimedon queenslandica ), the choanoflagellate M. brevicollis , the filasterean C. owczarzaki , three fungi ( Rhizopus oryzae, Laccaria bicolor and Neurospora crassa ), and the amoebozoan Dictyostelium discoideum . We also searched, if necessary, further basal eukaryotes whose genomes have been sequenced, in order to know the origin of gene families that could predate the split between amoebozoans and opisthokonts. Accession Codes : The whole genome sequence and annotated protein sequences of C. owczarzaki are deposited in NCBI with accession number ACFS01000000, BioProject ID PRJNA20341. The RNA-seq raw read sequences were submitted to NCBI’s Short Read Archive with the accession numbers SRX096928 , SRX096921 , SRX155797 , SRX155796 , SRX155795 , SRX155794 , SRX155793 , SRX155792 , SRX155791 , SRX155790 and SRX155789 . How to cite this article: Suga, H. et al . The Capsaspora genome reveals a complex unicellular prehistory of animals. Nat. Commun. 4:2325 doi: 10.1038/ncomms3325 (2013).